Prion protein facilitates uptake of zinc into neuronal cells Zinc is released into the synaptic cleft upon exocytotic stimuli, although the mechanism for its reuptake into neurons is unresolved. Here we show that the cellular prion protein enhances the uptake of zinc into neuronal cells. This prion-protein-mediated zinc influx requires the octapeptide repeats and amino-terminal polybasic region in the prion protein, but not its endocytosis. Selective antagonists of α-amino-3-hydroxy-5-methyl-4-isoxazolepropionate (AMPA) receptors block the prion protein-mediated zinc uptake, and the prion protein co-immunoprecipitates with both GluA1 and GluA2 AMPA receptor subunits. Zinc-sensitive intracellular tyrosine phosphatase activity is decreased in cells expressing prion protein and increased in the brains of prion-protein-null mice, providing evidence of a physiological consequence of this process. Prion protein-mediated zinc uptake is ablated in cells expressing familial associated mutants of the protein and in prion-infected cells. These data suggest that alterations in the cellular prion protein-mediated zinc uptake may contribute to neurodegeneration in prion and other neurodegenerative diseases. Zinc acts as a structural or catalytic component of a great number of proteins, and also functions as a neurotransmitter [1] . In addition, zinc modulates the function of glutamate and other neurotransmitter receptors [2] , and zinc is itself a signalling molecule directly regulating transcription factors [3] and inhibiting protein tyrosine phosphatases [4] , [5] . In neurons, zinc is packaged into synaptic vesicles alongside glutamate, and both are released into the synaptic cleft upon exocytotic stimuli [2] , [6] , [7] , [8] . The synaptically released zinc is then taken up into the cytoplasm of postsynaptic neurons, although the molecular mechanisms involved are far from clear [6] . In non-neuronal cells, the uptake of zinc across the plasma membrane is mediated by members of the ZIP (Zrt/Irt-like protein) family of zinc transporters [9] , whereas in neurons zinc enters through activated voltage-gated Ca 2+ channels, Ca 2+ and zinc-permeable α-amino-3-hydroxy-5-methyl-4-isoxazolepropionate (AMPA) receptors, and ZIP-1 and ZIP-3 (refs. 6 , 10 , 11 , 12 ). The intracellular zinc concentration is controlled by these zinc importers, along with zinc exporters (members of the ZnT/SLC30 family of transporters, which transport zinc from the cytosol to the lumen of intracellular organelles or out of the cell) and binding proteins such as metallothioneins [6] . Prion diseases such as the Creutzfeldt–Jakob disease (CJD) in humans are characterised by the conformational conversion of the cellular prion protein (PrP C ) into the protease-resistant, infectious form PrP Sc that aggregates in the brain [13] . Although the accumulation of PrP Sc is the main pathogenic event leading to neurodegeneration, loss of the normal function(s) of PrP C may also, in part, contribute to disease pathogenesis [14] , [15] . PrP C is a glycosyl-phosphatidylinositol-anchored protein located on the surface of neurons, at both pre- and postsynaptic sites, throughout the central nervous system and is particularly abundant in the hippocampus, frontal cortex and striatum [16] . Within the amino terminal half of the PrP C are four complete copies of the octapeptide repeat (PHGG(G/S)WGQ), which can bind copper and zinc [17] , [18] , [19] . Both copper and zinc, but not a range of other divalent metal ions, stimulate the endocytosis of PrP C (refs 20 , 21 ), and deletion of, or mutations within, the octapeptide repeats abrogate this metal-dependent endocytosis [20] . Studies using peptides encompassing the full metal-binding octapeptide repeats anchored to the surface of lipid vesicles have demonstrated that both copper and, more so, zinc promote PrP–PrP interactions, leading to the suggestion that PrP C may be capable of responding to fluctuations in neuronal zinc levels [22] . Recently, it was reported that prion genes are evolutionary descendants of the ZIP family of transmembrane zinc transporters [23] , adding further to our earlier proposal that PrP C may have a role in sensing, scavenging or transporting zinc from the extracellular milieu [24] . However, whether PrP C is indeed involved in zinc uptake, the molecular mechanism involved and the relevance of this to brain zinc homeostasis and neurodegeneration has yet to be determined. In this study, using two zinc-selective fluorescent dyes, Zinpyr-1 and Newport Green, we show for the first time that PrP C mediates the uptake of zinc into neuronal cells and that this uptake is mediated by AMPA receptors containing GluA1 and lacking GluA2 subunits. Zinc uptake is disrupted when PrP C is mutated or when cells are infected with prion, which suggests that the reduction in uptake of zinc contributes to the neurodegeneration that is commonly associated with prion diseases. PrP C enhances neuronal zinc uptake To investigate whether PrP C is involved in zinc uptake in neuronal cells, we exposed cells to zinc and measured the level of intracellular zinc using fluorescent dyes (Zinpyr-1 and Newport Green), which can be passively loaded into cells and used to detect intracellular-free (weakly bound, rapidly exchangeable) zinc. Untransfected SH-SY5Y cells, which do not endogenously express PrP C ( Fig. 1a insert) [20] , accumulated zinc in a dose-dependent manner as measured with Zinpyr-1 ( Fig. 1a ). However, SH-SY5Y cells stably expressing PrP C ( Fig. 1a insert) showed a significantly enhanced level of zinc-associated fluorescence ( Fig. 1a ). SH-SY5Y cells expressing PrP C also had a significantly enhanced rate of zinc uptake as measured kinetically using Newport Green as compared with the untransfected cells ( Fig. 1b ). The specificity of the Zinpyr-1 fluorescence for zinc was determined by incubation of SH-SY5Y cells expressing PrP C with other divalent cations (Mn 2+ , Fe 2+ , Ca 2+ or Cu 2+ ) before staining ( Fig. 1c ). Also, there was no competitive effect of either Cu 2+ or Mn 2+ when present in combination with zinc ( Fig. 1c ). Treatment with the zinc-specific chelators TPEN ( N,N,N,N -tetrakis(2-pyridylmethyl)ethylenediamine) or 1,10-phenanthroline before Zinpyr-1 staining resulted in a significant decrease in zinc-associated fluorescence, whereas exposure of the cells to the copper chelator bathocuproine sulphonate did not alter the Zinpyr-1 fluorescence ( Fig. 1d ), confirming the specificity of the Zinpyr-1 staining for zinc. Under the conditions used, zinc (at 32 μM or 100 μM) had no detrimental effect on the viability of the SH-SY5Y cells at any time point as measured by Hoecsht 33342 staining ( Supplementary Fig. S1a,b ) and the Promega Live/Dead assay (data not shown). 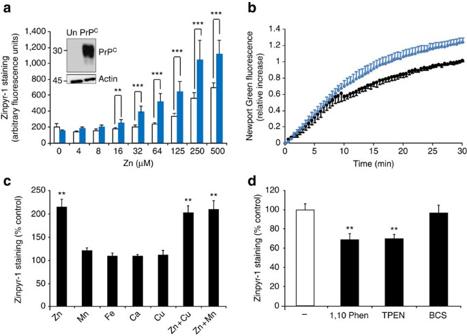Figure 1: PrPCselectively facilitates zinc uptake. (a) Untransfected SH-SY5Y cells (Un; white bars) or SH-SY5Y cells expressing PrPC(blue bars) were exposed to Zn2+for 6 h and then stained with 10 μM Zinpyr-1. Kruskal–Wallis, **P<0.01; ***P<0.001. Insert: detection of PrPCin the Un and PrPC-expressing cells with antibody 3F4, with actin as loading control. Molecular weight markers in kDa. (b) Kinetic analysis of the relative increase in zinc uptake using Newport Green in Un SH-SY5Y cells (black symbols) compared with SH-SY5Y cells expressing PrPC(blue symbols), exposed for up to 30 min to 32 μM Zn2+(n=3). Kruskal–Wallis,P<0.05. The specificity of the Zinpyr-1 staining was determined by exposure of the cells expressing PrPCto (c) alternative divalent cations (100 μM) or the indicated combinations, or (d) specific cation chelators (1,10-phenanthroline (1,10 Phen) 160 μM;N,N,N,N-tetrakis(2-pyridylmethyl)ethylenediamine (TPEN) 16 μM; bathocuproine sulphonate (BCS) 16 μM). Data shown as mean (±s.e.m.). Zinpyr-1 fluorescence corrected against DNA content (n=8). Kruskal–Wallis, **P<0.01. Figure 1: PrP C selectively facilitates zinc uptake. ( a ) Untransfected SH-SY5Y cells (Un; white bars) or SH-SY5Y cells expressing PrP C (blue bars) were exposed to Zn 2+ for 6 h and then stained with 10 μM Zinpyr-1. Kruskal–Wallis, ** P <0.01; *** P <0.001. Insert: detection of PrP C in the Un and PrP C -expressing cells with antibody 3F4, with actin as loading control. Molecular weight markers in kDa. ( b ) Kinetic analysis of the relative increase in zinc uptake using Newport Green in Un SH-SY5Y cells (black symbols) compared with SH-SY5Y cells expressing PrP C (blue symbols), exposed for up to 30 min to 32 μM Zn 2+ ( n =3). Kruskal–Wallis, P <0.05. The specificity of the Zinpyr-1 staining was determined by exposure of the cells expressing PrP C to ( c ) alternative divalent cations (100 μM) or the indicated combinations, or ( d ) specific cation chelators (1,10-phenanthroline (1,10 Phen) 160 μM; N,N,N,N -tetrakis(2-pyridylmethyl)ethylenediamine (TPEN) 16 μM; bathocuproine sulphonate (BCS) 16 μM). Data shown as mean (±s.e.m.). Zinpyr-1 fluorescence corrected against DNA content ( n =8). Kruskal–Wallis, ** P <0.01. Full size image To confirm a role for PrP C in enhancing zinc uptake in neuronal cells, both mouse N2a cells and rat primary hippocampal neurons were utilised in combination with small interfering RNA (siRNA) to knockdown endogenous PrP C and assess the effect of an acute loss of PrP C . Following siRNA treatment, there was a significant reduction (60±2%) in the amount of PrP C that could be detected in the N2a cells ( Fig. 2a insert), and zinc uptake was significantly suppressed as evaluated by both kinetic measurements ( Fig. 2a ) and fluorescence microscopy ( Fig. 2c ). In contrast, no alteration in zinc uptake was observed in the N2a cells treated with the non-targeting siRNA control ( Fig. 2b ). Immunofluorescence microscopy was used to validate the knockdown of PrP C in the hippocampal neurons ( Fig. 2d ). Zinc uptake was also reduced in hippocampal neurons treated with the PrP C -specific siRNA ( Fig. 2e ; Supplementary Fig. S2 ), but not in the neurons treated with the non-targeting siRNA control ( Fig. 2f ). Zinc (32 μM) did not decrease the viability of the N2a cells or the hippocampal neurons ( Supplementary Fig. S1c ). 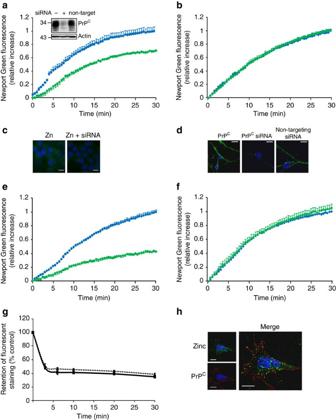Figure 2: PrPCfacilitates zinc uptake into neurons. Zinc uptake measured using Newport Green in N2a cells exposed for up to 30 min to (a) 32 μM Zn2+(blue symbols) or to 32 μM Zn2+following knockdown of PrPCwith siRNA (green symbols; Kruskal–Wallis,P<0.05) or to (b) 32 μM Zn2+(blue symbols) or 32 μM Zn2+with non-targeting siRNA control (green symbols;n=6). Insert ina: expression of PrPCin untreated, PrPC-specific siRNA or non-targeting siRNA-treated N2a cells, with actin as loading control. (c) Zinc uptake visualised by fluorescence microscopy using Newport Green in N2a cells exposed to 100 μM Zn2+(Zn) or to 100 μM Zn2+following knockdown of PrPCexpression with siRNA (Zn+siRNA). Scale bars equal 10 μm. (d) Fluorescence images of primary hippocampal neurons showing the distribution of PrPC(probed with antibody 6H4) in untreated, PrPC-specific siRNA-treated or non-targeting siRNA-treated cells. Scale bar equals 10 μm (n=10). Zinc uptake measured using Newport Green in rat primary hippocampal neurons exposed for up to 30 min to (e) 32 μM Zn2+(blue symbols) or to 32 μM Zn2+following knockdown of PrPCexpression with siRNA (green symbols; Kruskal–Wallis,P<0.05) or to (f) 32 μM Zn2+(blue symbols) or 32 μM Zn2+with non-targeting siRNA control (green symbols;n=3). Data shown as the relative Newport Green fluorescence corrected against DNA content and plotted as mean±s.e.m. (g) Untransfected SH-SY5Y cells (dotted line) or SH-SY5Y cells expressing PrPC(solid line) were pre-loaded with 32 μM Zn, followed by 5 μM Newport Green for a further 30 min, to label the intracellular Zn. The change in fluorescence with time was measured on addition of fresh medium to determine whether PrPCpromoted retention of Zn. (h) Cellular localisation of Newport Green fluorescence (green) and PrPC(red) in SH-SY5Y cells expressing PrPCexposed to 32 μM Zn. Scale bars equal 5 μm. Figure 2: PrP C facilitates zinc uptake into neurons. Zinc uptake measured using Newport Green in N2a cells exposed for up to 30 min to ( a ) 32 μM Zn 2+ (blue symbols) or to 32 μM Zn 2+ following knockdown of PrP C with siRNA (green symbols; Kruskal–Wallis, P <0.05) or to ( b ) 32 μM Zn 2+ (blue symbols) or 32 μM Zn 2+ with non-targeting siRNA control (green symbols; n =6). Insert in a : expression of PrP C in untreated, PrP C -specific siRNA or non-targeting siRNA-treated N2a cells, with actin as loading control. ( c ) Zinc uptake visualised by fluorescence microscopy using Newport Green in N2a cells exposed to 100 μM Zn 2+ (Zn) or to 100 μM Zn 2+ following knockdown of PrP C expression with siRNA (Zn+siRNA). Scale bars equal 10 μm. ( d ) Fluorescence images of primary hippocampal neurons showing the distribution of PrP C (probed with antibody 6H4) in untreated, PrP C -specific siRNA-treated or non-targeting siRNA-treated cells. Scale bar equals 10 μm ( n =10). Zinc uptake measured using Newport Green in rat primary hippocampal neurons exposed for up to 30 min to ( e ) 32 μM Zn 2+ (blue symbols) or to 32 μM Zn 2+ following knockdown of PrP C expression with siRNA (green symbols; Kruskal–Wallis, P <0.05) or to ( f ) 32 μM Zn 2+ (blue symbols) or 32 μM Zn 2+ with non-targeting siRNA control (green symbols; n =3). Data shown as the relative Newport Green fluorescence corrected against DNA content and plotted as mean±s.e.m. ( g ) Untransfected SH-SY5Y cells (dotted line) or SH-SY5Y cells expressing PrP C (solid line) were pre-loaded with 32 μM Zn, followed by 5 μM Newport Green for a further 30 min, to label the intracellular Zn. The change in fluorescence with time was measured on addition of fresh medium to determine whether PrP C promoted retention of Zn. ( h ) Cellular localisation of Newport Green fluorescence (green) and PrP C (red) in SH-SY5Y cells expressing PrP C exposed to 32 μM Zn. Scale bars equal 5 μm. Full size image To exclude the possibility that PrP C was enhancing retention of zinc within the cell rather than increasing its uptake, untransfected SH-SY5Y cells and cells expressing PrP C were preloaded with zinc before the addition of Newport Green, and then the change in fluorescence was measured over time. As the zinc was transported out of the cells, there was a reduction in fluorescence over time; however, there was no difference in the rate by which the fluorescence changed between the untransfected and PrP C -expressing cells ( Fig. 2g ). Fluorescence microscopy of permeabilised cells revealed virtually no overlap in the distribution of PrP C and the Newport-Green staining for zinc ( Fig. 2h ). The punctuate staining for zinc reflects the way in which it is stored, as very little zinc exists free in the cytosol. Rather it is stored in at least three pools: tightly bound to a wide variety of proteins, bound to metallothioneins or accumulated in the lumen of cytoplasmic vesicles and organelles [27] . These data, together with the fact that PrP C is located on the outer surface of the plasma membrane or in the lumen of the secretory pathway, whereas the Newport-Green staining for zinc is predominantly in the cytosol, indicates that PrP C is not acting to directly sequester zinc inside the cell. In contrast to PrP C , the sequence-related proteins Shadoo and Doppel did not enhance the uptake of zinc into the SH-SY5Y cells ( Fig. 3a,b ). Together, these data, using two different zinc-selective dyes and multiple cell systems, demonstrate for the first time that PrP C selectively enhances zinc uptake into neuronal cells. 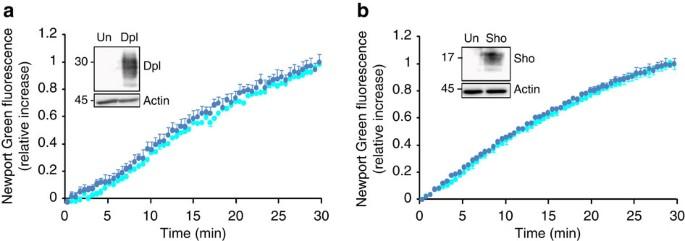Figure 3: Neither Doppel (Dpl) nor Shadoo (Sho) facilitate zinc uptake. Zinc uptake measured using Newport Green in SH-SY5Y cells expressing (a) Dpl or (b) Sho, either not supplemented with Zn2+(light blue symbols) or supplemented with 32 μM Zn2+(dark blue symbols). Data shown as the relative Newport Green fluorescence corrected against DNA content and are representative of six independent experiments. Inserts show the expression of (a) Dpl or (b) Sho in the SH-SY5Y cells as detected by western blotting with DDC39 (Dpl) or anti-Sho antibodies (equal protein loading shown by detection of actin). Molecular weight markers in kDa. Un, untransfected. Figure 3: Neither Doppel (Dpl) nor Shadoo (Sho) facilitate zinc uptake. Zinc uptake measured using Newport Green in SH-SY5Y cells expressing ( a ) Dpl or ( b ) Sho, either not supplemented with Zn 2+ (light blue symbols) or supplemented with 32 μM Zn 2+ (dark blue symbols). Data shown as the relative Newport Green fluorescence corrected against DNA content and are representative of six independent experiments. Inserts show the expression of ( a ) Dpl or ( b ) Sho in the SH-SY5Y cells as detected by western blotting with DDC39 (Dpl) or anti-Sho antibodies (equal protein loading shown by detection of actin). Molecular weight markers in kDa. Un, untransfected. Full size image The uptake of zinc does not require the endocytosis of PrP C As zinc promotes the endocytosis of PrP C (ref. 20 ), we investigated whether the increase in intracellular zinc required the endocytosis of the protein. The copper-mediated endocytosis of PrP C in SH-SY5Y cells is dependent on the transmembrane low-density lipoprotein receptor-related protein-1 (LRP1) [28] . First, to ascertain whether the zinc-mediated endocytosis of PrP C was also dependent on LRP1, we used soluble receptor-associated protein (RAP) to inhibit the interaction between the two proteins and siRNA knockdown of LRP1 in conjunction with the established endocytosis assay involving surface biotinylation and trypsin digestion [28] . Co-incubation of the cells with RAP during the zinc incubation period significantly inhibited the endocytosis of PrP C , as did the siRNA-mediated knockdown of LRP1 before the addition of zinc ( Fig. 4a and b ), indicating that the zinc-mediated endocytosis of PrP C is also dependent on LRP1. However, blocking the endocytosis of PrP C either by siRNA knockdown of LRP1 ( Fig. 4c ) or with RAP ( Fig. 4d ) did not reduce the uptake of zinc into the cells, indicating that the endocytosis of PrP C is not the mechanism responsible for the enhanced uptake of zinc. Interestingly, both RAP and siRNA knockdown of LRP1 caused a small but significant increase in the uptake of zinc ( Fig. 4c and d ). It is possible that blocking the endocytosis of PrP C would cause more PrP C to be available at the cell surface to facilitate zinc uptake. 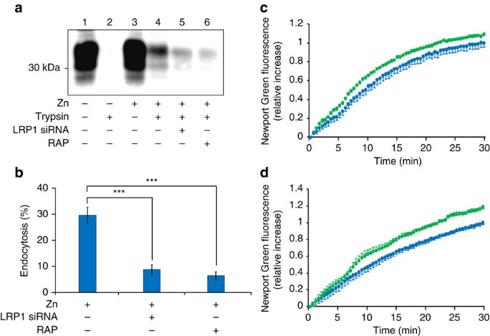Figure 4: Zinc uptake does not require the endocytosis of PrPC. (a) SH-SY5Y cells expressing PrPCwere surface biotinylated and then either left untreated, exposed to 20 μg ml−1RAP or 2 μM LRP1 siRNA in the presence or absence of 100 μM Zn2+. Before lysis, cell-surface PrPCwas removed by trypsin digestion. PrPCwas immunoprecipitated from the cell lysates with antibody 3F4 and analysed by western blot with the biotin-labelled PrPCdetected with peroxidase-conjugated streptavidin. (b) Quantification of the inhibitory effect of RAP and LRP1 siRNA treatment on the amount of zinc-stimulated endocytosis across multiple immunoblots from three separate experiments. Kruskal–Wallis, ***P<0.001. (c) Zinc uptake measured using Newport Green in SH-SY5Y cells expressing PrPCexposed to 100 μM Zn2+(blue symbols) or to 100 μM Zn2+following knockdown of LRP1 expression with siRNA (green symbols). Kruskal–Wallis,P<0.05. (d) Zinc uptake measured using Newport Green in SH-SY5Y cells expressing PrPCexposed to 100 μM Zn2+(blue symbols) or to 100 μM Zn2+in the presence of 20 μg ml−1RAP (green symbols). Kruskal–Wallis,P<0.05. Data shown as the relative Newport Green fluorescence corrected against DNA content and plotted as mean±s.e.m. (n=3). Figure 4: Zinc uptake does not require the endocytosis of PrP C . ( a ) SH-SY5Y cells expressing PrP C were surface biotinylated and then either left untreated, exposed to 20 μg ml −1 RAP or 2 μM LRP1 siRNA in the presence or absence of 100 μM Zn 2+ . Before lysis, cell-surface PrP C was removed by trypsin digestion. PrP C was immunoprecipitated from the cell lysates with antibody 3F4 and analysed by western blot with the biotin-labelled PrP C detected with peroxidase-conjugated streptavidin. ( b ) Quantification of the inhibitory effect of RAP and LRP1 siRNA treatment on the amount of zinc-stimulated endocytosis across multiple immunoblots from three separate experiments. Kruskal–Wallis, *** P <0.001. ( c ) Zinc uptake measured using Newport Green in SH-SY5Y cells expressing PrP C exposed to 100 μM Zn 2+ (blue symbols) or to 100 μM Zn 2+ following knockdown of LRP1 expression with siRNA (green symbols). Kruskal–Wallis, P <0.05. ( d ) Zinc uptake measured using Newport Green in SH-SY5Y cells expressing PrP C exposed to 100 μM Zn 2+ (blue symbols) or to 100 μM Zn 2+ in the presence of 20 μg ml −1 RAP (green symbols). Kruskal–Wallis, P <0.05. Data shown as the relative Newport Green fluorescence corrected against DNA content and plotted as mean±s.e.m. ( n =3). Full size image The PrP C -enhanced zinc uptake is mediated by AMPA receptors Having excluded PrP C endocytosis as the mechanism behind the enhanced uptake of zinc, we investigated alternative routes by which zinc may be entering the cells. It has been shown previously that zinc can enter neurons through AMPA receptors [10] . To investigate whether AMPA receptors were involved in the PrP C -mediated zinc uptake, the SH-SY5Y cells were incubated with CNQX, a competitive AMPA/kainate receptor antagonist. CNQX significantly reduced the uptake of zinc in the cells expressing PrP C ( Fig. 5a ), but had no effect on the uptake of zinc in the untransfected cells ( Fig. 5b ). The ability of CNQX to reduce the PrP C -enhanced uptake of zinc was confirmed by immunofluorescence microscopy of the cells following exposure to Newport Green ( Fig. 5c ). CNQX also significantly reduced the uptake of zinc into the hippocampal neurons to a level similar to that observed following knockdown of PrP C expression by siRNA ( Fig. 5d ). Indeed, when the two treatments were combined, addition of CNQX did not further decrease zinc uptake beyond that observed for the siRNA knockdown of PrP C ( Fig. 5e ). We also explored the effect of direct activation of AMPA receptors on zinc uptake. The siRNA knockdown of PrP C in the hippocampal neurons ablated the AMPA-mediated increase in zinc uptake ( Fig. 5f ). Together, these data suggest that the PrP C -enhanced zinc uptake is mediated by AMPA receptors. 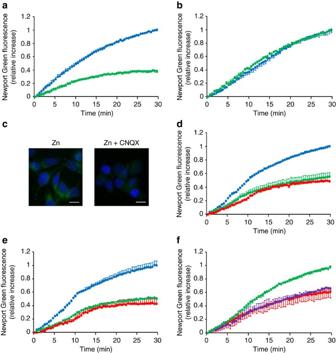Figure 5: PrPC-enhanced zinc uptake requires AMPA receptors. Zinc uptake measured using Newport Green in (a) SH-SY5Y cells expressing PrPCor in (b) untransfected SH-SY5Y cells exposed to 32 μM Zn2+(blue symbols) or to 32 μM Zn2+and 10 μM CNQX (green symbols). Kruskal–Wallis,P<0.05 ina. (c) Zinc uptake visualised using Newport Green in SH-SY5Y cells expressing PrPCexposed to 32 μM Zn2+or to 32 μM Zn2+in the presence of 10 μM CNQX. Scale bars equal 10 μm. (d) Zinc uptake measured using Newport Green in rat primary hippocampal neurons exposed to 32 μM Zn2+(blue symbols), to 32 μM Zn2+and 10 μM CNQX (green symbols), or to 32 μM Zn2+following knockdown of PrPCexpression with siRNA (red symbols). (e) Zinc uptake measured using Newport Green in rat primary hippocampal neurons exposed to 32 μM Zn2+(blue symbols) or to 32 μM Zn2+following knockdown of PrPCexpression with siRNA (green symbols), or 32 μM Zn2+and 10 μM CNQX following knockdown of PrPCexpression with siRNA (red symbols). (f) Zinc uptake measured using Newport Green in rat primary hippocampal neurons exposed to 32 μM Zn2+in the presence of 100 μM AMPA (green symbols) following knockdown of PrPCexpression with siRNA (red symbols), or to 100 μM AMPA following knockdown of PrPCexpression with siRNA (purple symbols). Data shown as the relative Newport Green fluorescence corrected against DNA content and plotted as mean±s.e.m. (n=3). Figure 5: PrP C -enhanced zinc uptake requires AMPA receptors. Zinc uptake measured using Newport Green in ( a ) SH-SY5Y cells expressing PrP C or in ( b ) untransfected SH-SY5Y cells exposed to 32 μM Zn 2+ (blue symbols) or to 32 μM Zn 2+ and 10 μM CNQX (green symbols). Kruskal–Wallis, P <0.05 in a . ( c ) Zinc uptake visualised using Newport Green in SH-SY5Y cells expressing PrP C exposed to 32 μM Zn 2+ or to 32 μM Zn 2+ in the presence of 10 μM CNQX. Scale bars equal 10 μm. ( d ) Zinc uptake measured using Newport Green in rat primary hippocampal neurons exposed to 32 μM Zn 2+ (blue symbols), to 32 μM Zn 2+ and 10 μM CNQX (green symbols), or to 32 μM Zn 2+ following knockdown of PrP C expression with siRNA (red symbols). ( e ) Zinc uptake measured using Newport Green in rat primary hippocampal neurons exposed to 32 μM Zn 2+ (blue symbols) or to 32 μM Zn 2+ following knockdown of PrP C expression with siRNA (green symbols), or 32 μM Zn 2+ and 10 μM CNQX following knockdown of PrP C expression with siRNA (red symbols). ( f ) Zinc uptake measured using Newport Green in rat primary hippocampal neurons exposed to 32 μM Zn 2+ in the presence of 100 μM AMPA (green symbols) following knockdown of PrP C expression with siRNA (red symbols), or to 100 μM AMPA following knockdown of PrP C expression with siRNA (purple symbols). Data shown as the relative Newport Green fluorescence corrected against DNA content and plotted as mean±s.e.m. ( n =3). Full size image Mechanism of PrP C -mediated zinc uptake via AMPA receptors To characterise further the role of AMPA receptors in the PrP C -enhanced zinc uptake, the Newport-Green fluorescence was measured in the SH-SY5Y cells expressing PrP C and in the hippocampal neurons exposed to either IEM-1460 or pentobarbital, which inhibit GluA2-lacking or GluA2-containing AMPA receptors, respectively. Surprisingly, both IEM-1460 ( Fig. 6a,b ) and pentobarbital ( Fig. 6c,d ) diminished the PrP C -mediated zinc uptake. Previously, PrP C has been shown to interact with the GluA2 subunit of AMPA receptors [29] . To confirm this observation and to determine whether PrP C also interacts with the GluA1 subunit, immunoprecipitation from mouse brain homogenate using antibodies against PrP C , GluA1 and GluA2 was performed and the resulting immunoprecipitates western blotted with antibodies against each protein. Both GluA1 and GluA2 co-immunoprecipitated with PrP C , and PrP C co-immunoprecipitated with both GluA1 and GluA2 ( Fig. 6e ). No co-immunoprecipitation was observed using Sepharose beads only, or with beads coated with a non-specific IgG ( Fig. 6e ) or using brain homogenate from a PrP-null mouse ( Fig. 6f ). In addition, PrP C increased the cell surface expression of the GluA1 subunit ( Fig. 6g,h ). 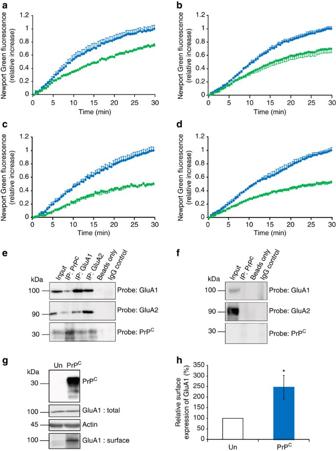Figure 6: PrPCinteracts with AMPA receptor subunits. Zinc uptake measured using Newport Green in SH-SY5Y cells expressing PrPC(a,c) and in rat primary hippocampal neurons (b,d) exposed to 32 μM Zn2+(blue symbols) or to 32 μM Zn2+, and (a,b) 10 μM IEM-1460 (green symbols) or (c,d) 100 μM pentobarbital (green symbols). Data shown as the relative Newport Green fluorescence corrected against DNA content and plotted as mean±s.e.m. (n=3). Kruskal–Wallis,P<0.05. Co-immunoprecipitation from (e) wild-type 129/P2 or (f) PrP−/−129/P2 mouse brain using antibodies against PrPC(6H4), GluA1, GluA2, control rabbit anti-mouse IgG or no antibody for the bead-only control, and then probed with antibodies against PrPC(SAF32), GluA1 or GluA2 as indicated. (g) Cell lysates from either untransfected (Un) SH-SY5Y cells or those expressing PrPCwere analysed for their expression of PrPCand GluA1. Actin was included as a loading control. Cell monolayers were treated with cell-impermeant biotin to determine the amount of GluA1 at the cell surface. GluA1 was immunoprecipitated from the lysates and the biotin-labelled GluA1 detected using peroxidase-conjugated streptavidin. (h) Cell surface GluA1 was quantified from multiple immunoblots (n=3). Kruskal–Wallis, *P<0.05. Figure 6: PrP C interacts with AMPA receptor subunits. Zinc uptake measured using Newport Green in SH-SY5Y cells expressing PrP C ( a , c ) and in rat primary hippocampal neurons ( b , d ) exposed to 32 μM Zn 2+ (blue symbols) or to 32 μM Zn 2+ , and ( a , b ) 10 μM IEM-1460 (green symbols) or ( c , d ) 100 μM pentobarbital (green symbols). Data shown as the relative Newport Green fluorescence corrected against DNA content and plotted as mean±s.e.m. ( n =3). Kruskal–Wallis, P <0.05. Co-immunoprecipitation from ( e ) wild-type 129/P2 or ( f ) PrP −/− 129/P2 mouse brain using antibodies against PrP C (6H4), GluA1, GluA2, control rabbit anti-mouse IgG or no antibody for the bead-only control, and then probed with antibodies against PrP C (SAF32), GluA1 or GluA2 as indicated. ( g ) Cell lysates from either untransfected (Un) SH-SY5Y cells or those expressing PrP C were analysed for their expression of PrP C and GluA1. Actin was included as a loading control. Cell monolayers were treated with cell-impermeant biotin to determine the amount of GluA1 at the cell surface. GluA1 was immunoprecipitated from the lysates and the biotin-labelled GluA1 detected using peroxidase-conjugated streptavidin. ( h ) Cell surface GluA1 was quantified from multiple immunoblots ( n =3). Kruskal–Wallis, * P <0.05. Full size image To explore further the molecular mechanism underlying the PrP C -mediated zinc uptake via AMPA receptors, we determined the regions of PrP C involved in (i) the uptake of zinc and (ii) the interaction with AMPA receptors. Cells expressing wild-type PrP C were incubated with epitope-specific antibodies before exposure to zinc. Incubation of the cells with antibody SAF32, which recognises an epitope encompassing amino acids 59–89 contained within the octapeptide repeat region, significantly reduced the uptake of zinc ( Fig. 7a ), whereas incubation of the cells with antibody 8H4, which recognises residues 175–185, had no effect on the PrP C -mediated increase in zinc uptake ( Fig. 7a ). Incubation of the cells with a non-specific antibody (against the transferrin receptor) had no effect on the uptake of zinc ( Fig. 7a ). Antibody SAF32, but not the transferrin-receptor antibody, also significantly reduced the uptake of zinc in the hippocampal neurons ( Fig. 7b ). To explore further the role of the metal-binding octapeptide repeats of PrP C in the uptake of zinc, we utilised cells expressing PrPΔOct, in which the octapeptide repeat sequence has been removed [20] . The Zinpyr-1 fluorescence in the SH-SY5Y cells expressing PrPΔOct ( Fig. 7c insert) following exposure to zinc was similar to that of the untransfected cells ( Fig. 7c ). Next, we investigated whether the octapeptide repeats were required for the interaction with AMPA receptors. PrPΔOct still co-immunoprecipitated with the GluA2 subunit ( Fig. 7d ), and wild-type PrP C co-immunoprecipiated with both GluA1 and GluA2 following chelation of zinc ( Fig. 7e ). To explore further the region of PrP C involved in the interaction with the AMPA receptor, we utilised a construct of PrP C , PrPΔN, which lacks the four amino acids (lysyl-lysyl-arginyl-proline) from the N terminus of the mature protein [30] . PrPΔN is trafficked to the cell surface, localised to detergent-resistant lipid rafts and undergoes endoproteolytic cleavage to generate the C1 fragment similarly to wild-type PrP C (refs 30 , 31 , 32 ). However, PrPΔN failed to enhance the uptake of zinc into cells ( Fig. 7c ) and also failed to co-immunoprecipitate with the GluA2 subunit ( Fig. 7d ). These data indicate that the metal-binding octapeptide repeats in PrP C are required for the enhanced zinc uptake but not for the interaction with the AMPA receptor, whereas the N-terminal polybasic region of the protein is critical for the interaction with the AMPA receptor. 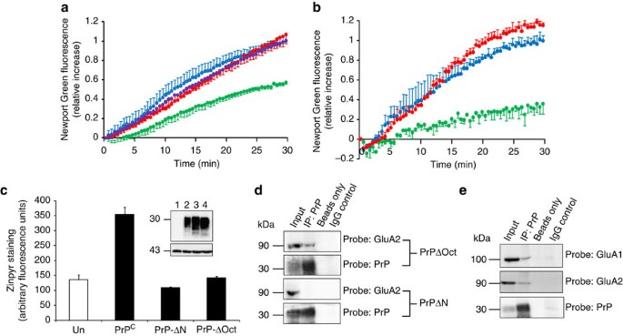Figure 7: The N terminus of PrPCis required for the interaction with AMPA subunits. (a) Zinc uptake measured using Newport Green in SH-SY5Y cells expressing wild-type PrPCexposed to 32 μM Zn2+(blue symbols), 32 μM Zn2+and 10 μg ml−1antibody SAF32 (green symbols), 32 μM Zn2+and 10 μg ml−1antibody 8H4 (red symbols) or 32 μM Zn2+and 10 μg ml−1anti-transferrin receptor antibody (purple symbols). (b) Zinc uptake measured using Newport Green in rat primary hippocampal neurons exposed to 32 μM Zn2+(blue symbols), 32 μM Zn2+and 10 μg ml−1antibody SAF32 (green symbols) or 32 μM Zn2+and 10 μg ml−1anti-transferrin receptor antibody (red symbols). Data shown as the relative Newport Green fluorescence corrected against DNA content and are plotted as mean±s.e.m. (n=3). Kruskal–Wallis,P<0.05 for SAF32 compared with no antibody. (c) Untransfected (Un) SH-SY5Y cells or SH-SY5Y cells expressing either wild-type PrPC, PrPΔOct or PrPΔN were exposed to 100 μM Zn2+and stained using 10 μM Zinpyr-1. Data shown as mean (±s.e.m.). Zinpyr-1 fluorescence corrected against DNA content (n=8). Insert shows expression of wild-type PrPC, PrPΔOct and PrPΔN with actin as a loading control. Molecular weight markers in kDa. (d) Co-immunoprecipitation from lysates of SH-SY5Y cells expressing PrPΔOct or PrPΔN using antibodies against PrPC(6H4), GluA2, control rabbit anti-mouse IgG or no antibody for the bead-only control, and then probed with antibodies against PrPC(6D11 for PrPΔOct or SAF32 for PrPΔN) or GluA2 as indicated. (e) Co-immunoprecipitation from wild-type Ola/P2 mouse brain using antibodies against PrPC(6H4), GluA1, GluA2, control rabbit anti-mouse IgG or no antibody for the bead-only control with 20 μM TPEN included in all buffers and washes. Samples were probed with antibodies against PrPC(SAF32), GluA1 or GluA2 as indicated. Figure 7: The N terminus of PrP C is required for the interaction with AMPA subunits. ( a ) Zinc uptake measured using Newport Green in SH-SY5Y cells expressing wild-type PrP C exposed to 32 μM Zn 2+ (blue symbols), 32 μM Zn 2+ and 10 μg ml −1 antibody SAF32 (green symbols), 32 μM Zn 2+ and 10 μg ml −1 antibody 8H4 (red symbols) or 32 μM Zn 2+ and 10 μg ml −1 anti-transferrin receptor antibody (purple symbols). ( b ) Zinc uptake measured using Newport Green in rat primary hippocampal neurons exposed to 32 μM Zn 2+ (blue symbols), 32 μM Zn 2+ and 10 μg ml −1 antibody SAF32 (green symbols) or 32 μM Zn 2+ and 10 μg ml −1 anti-transferrin receptor antibody (red symbols). Data shown as the relative Newport Green fluorescence corrected against DNA content and are plotted as mean±s.e.m. ( n =3). Kruskal–Wallis, P <0.05 for SAF32 compared with no antibody. ( c ) Untransfected (Un) SH-SY5Y cells or SH-SY5Y cells expressing either wild-type PrP C , PrPΔOct or PrPΔN were exposed to 100 μM Zn 2+ and stained using 10 μM Zinpyr-1. Data shown as mean (±s.e.m.). Zinpyr-1 fluorescence corrected against DNA content ( n =8). Insert shows expression of wild-type PrP C , PrPΔOct and PrPΔN with actin as a loading control. Molecular weight markers in kDa. ( d ) Co-immunoprecipitation from lysates of SH-SY5Y cells expressing PrPΔOct or PrPΔN using antibodies against PrP C (6H4), GluA2, control rabbit anti-mouse IgG or no antibody for the bead-only control, and then probed with antibodies against PrP C (6D11 for PrPΔOct or SAF32 for PrPΔN) or GluA2 as indicated. ( e ) Co-immunoprecipitation from wild-type Ola/P2 mouse brain using antibodies against PrP C (6H4), GluA1, GluA2, control rabbit anti-mouse IgG or no antibody for the bead-only control with 20 μM TPEN included in all buffers and washes. Samples were probed with antibodies against PrP C (SAF32), GluA1 or GluA2 as indicated. Full size image Tyrosine phosphatase activity is increased in PrP C -null mice Intracellular protein tyrosine phosphatase activity is exquisitely sensitive to zinc [4] , [5] . Therefore, to determine whether the increased uptake of zinc observed in cells expressing PrP C affected a cellular event, we measured the tyrosine phosphatase activity in the cells. In agreement with previous reports [4] , [5] , zinc directly inhibited phosphatase activity when added to the SH-SY5Y cell lysate ( Supplementary Fig. S3 ). In the cells expressing PrP C , there was a significant reduction of phosphatase activity as compared with the untransfected cells ( Fig. 8a ), indicating that the enhanced uptake of zinc by PrP C has a downstream effect on a cellular process. To confirm that PrP C disrupted zinc homeostasis in vivo , we measured the tyrosine phosphatase activity in the brains of wild-type and PrP C -null mice. Consistent with a role for PrP C in neuronal zinc uptake, there was a higher level of tyrosine phosphatase activity in the brains of the PrP C -null mice compared with the wild-type, age-matched control mice ( Fig. 8b ). These data, for the first time, indicate that PrP C is involved in the physiological homeostasis of neuronal zinc. 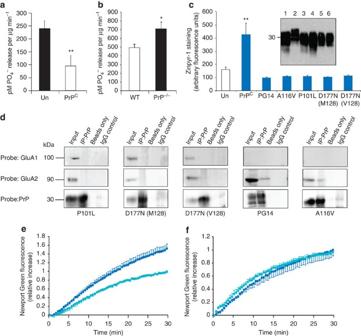Figure 8: Protein tyrosine phosphatase activity is enhanced in PrPC-null mice and zinc uptake is reduced in prion disease. (a) Lysates from untransfected SH-SY5Y cells (Un) or cells expressing PrPCwere incubated with phosphopeptide for 45 min at 37 °C to measure tyrosine phosphatase activity. Data shown as mean (±s.e.m.) (n=3). Independent Student'st-test, **P<0.01. (b) Tyrosine phosphatase activity was measured in whole-brain homogenate from wild-type 129/P2 (WT) or 129/P2 PrP−/−mice. Data shown as mean (±s.e.m.;n=8). Independent Student'st-test, *P<0.05. (c) SH-SY5Y cells expressing the various disease-associated mutants of PrPCwere exposed to 100 μM Zn2+and stained using 10 μM Zinpyr-1. Data shown as mean (±s.e.m.). Zinpyr-1 fluorescence corrected against DNA content (n=8). Kruskal–Wallis, **P<0.01. Insert shows expression of the various disease-associated mutants of PrPC. Lane 1, wild-type PrPC; lane 2, PG14; lane 3, A116V; lane 4, P101L; lane 5, D177N/M128; and lane 6, D117N/V128. Molecular weight marker in kDa. (d) Co-immunoprecipitation from P101 L, D177N (M128), D177N (V128) mouse brain or SH-SY5Y cell lysates expressing PG14 or A116V using antibodies against PrPC(6H4), control rabbit anti-mouse IgG or no antibody for the bead-only control, and then probed with antibodies against PrPC(SAF32), GluA1 or GluA2 as indicated. Zinc uptake measured using Newport Green in (e) uninfected N2a cells and (f) scrapie-infected ScN2a cells, either not supplemented with Zn2+(light blue symbols) or supplemented with 32 μM Zn2+(dark blue symbols). Data shown as the relative Newport Green fluorescence corrected against DNA content and plotted as mean±s.e.m. (n=3). Kruskal–Wallis,P<0.05 in the uninfected cells. Figure 8: Protein tyrosine phosphatase activity is enhanced in PrP C -null mice and zinc uptake is reduced in prion disease. ( a ) Lysates from untransfected SH-SY5Y cells (Un) or cells expressing PrP C were incubated with phosphopeptide for 45 min at 37 °C to measure tyrosine phosphatase activity. Data shown as mean (±s.e.m.) ( n =3). Independent Student's t -test, ** P <0.01. ( b ) Tyrosine phosphatase activity was measured in whole-brain homogenate from wild-type 129/P2 (WT) or 129/P2 PrP −/− mice. Data shown as mean (±s.e.m. ; n =8). Independent Student's t -test, * P <0.05. ( c ) SH-SY5Y cells expressing the various disease-associated mutants of PrP C were exposed to 100 μM Zn 2+ and stained using 10 μM Zinpyr-1. Data shown as mean (±s.e.m.). Zinpyr-1 fluorescence corrected against DNA content ( n =8). Kruskal–Wallis, ** P <0.01. Insert shows expression of the various disease-associated mutants of PrP C . Lane 1, wild-type PrP C ; lane 2, PG14; lane 3, A116V; lane 4, P101L; lane 5, D177N/M128; and lane 6, D117N/V128. Molecular weight marker in kDa. ( d ) Co-immunoprecipitation from P101 L, D177N (M128), D177N (V128) mouse brain or SH-SY5Y cell lysates expressing PG14 or A116V using antibodies against PrP C (6H4), control rabbit anti-mouse IgG or no antibody for the bead-only control, and then probed with antibodies against PrP C (SAF32), GluA1 or GluA2 as indicated. Zinc uptake measured using Newport Green in ( e ) uninfected N2a cells and ( f ) scrapie-infected ScN2a cells, either not supplemented with Zn 2+ (light blue symbols) or supplemented with 32 μM Zn 2+ (dark blue symbols). Data shown as the relative Newport Green fluorescence corrected against DNA content and plotted as mean±s.e.m. ( n =3). Kruskal–Wallis, P <0.05 in the uninfected cells. Full size image Enhanced uptake of zinc is lost in prion disease As zinc is reduced in the brain in prion disease [33] , [34] , and there is debate whether prion diseases involve a loss of a normal function of PrP C in addition to the toxic gain-of-function [14] , [15] , we investigated the effect of a number of prion disease-associated mutations in PrP C on zinc uptake. PG14 has an additional nine octapeptide repeats and results in familial CJD [35] , whereas A116V and P101L are both single point mutations, which cause the Gerstmann–Straussler–Scheinker syndrome (GSS) [36] , [37] . D177N with valine at position 128 (D177N/V128) also results in GSS, whereas with methionine at position 128 (D177N/M128) causes familial fatal insomnia [38] . All mutants were stably expressed in SH-SY5Y cells to similar levels ( Fig. 8c insert). In contrast to wild-type PrP C , none of the five disease-associated mutants of PrP C enhanced zinc uptake above that seen in the untransfected cells ( Fig. 8c ). To investigate the mechanism underlying the lack of zinc uptake in the disease-associated mutants of PrP C , we determined whether they co-immunoprecipitated with the AMPA receptor. Neither of the D177N mutants nor P101L interacted with the GluA1 or GluA2 subunits ( Fig. 8d ), indicating that in these disease-associated mutants of PrP C the mechanism underlying the inability to enhance zinc uptake may be due to loss of the interaction with AMPA receptors. Although the PG14 and A116V mutants still co-immunoprecipitated with the GluA2 subunit, in the cells expressing these two mutants we observed that the level of the GluA1 subunit was significantly reduced ( Fig. 8d and Supplementary Fig. S4 ), suggesting that this likely underlies the inability of the PG14 and A116V mutants to increase zinc uptake. Finally, to determine whether zinc uptake was affected upon the conformational conversion of PrP C to PrP Sc , zinc uptake was measured in persistently scrapie-infected ScN2a cells. Although a significant increase in zinc uptake was measured in uninfected N2a cells following exposure to exogenous zinc ( Fig. 8e ), no such increase was measured in the scrapie-infected ScN2a cells ( Fig. 8f ). These data indicate that the PrP C -mediated zinc uptake is lost in cells expressing prion disease-associated mutants of PrP C and upon conversion of PrP C to PrP Sc . Zinc can bind to the octapeptide repeats in PrP C (refs 18 , 19 , 22 ) and promote its endocytosis [20] , [21] ; however, the role of PrP C in cellular zinc metabolism has remained enigmatic. For the first time, by utilising zinc-specific fluorescent dyes, we have shown that PrP C via AMPA receptors directly influences the zinc content of neuronal cells. We have also shown that the role of PrP C in neuronal zinc homeostasis is of functional relevance, as evidenced by the increase in intracellular zinc-sensitive protein tyrosine phosphatase activity in the brains of PrP C -null mice. Our observations are consistent with, and provide the first mechanistic explanation for, the recent reports of reduced zinc in the hippocampus and other brain regions of PrP C -null mice [39] and of altered levels of zinc in specific brain regions of PrP C transgenic mice [39] . Our data suggest that PrP C may provide neuroprotection by facilitating the reuptake of the potentially neurotoxic synaptic zinc released upon glutamatergic neurotransmission. Furthermore, by reduction of protein tyrosine phosphatase activity, this PrP C -mediated increase in intracellular zinc may affect learning and memory [40] , and promote neuronal survival [41] . Our data show that PrP C enhances zinc uptake through AMPA receptors, which are known to have a key role in zinc homeostasis in neurons [6] . AMPA receptors are composed of various combinations of four subunits (GluA1–GluA4) and are widely expressed in neurons throughout the central nervous system. In the hippocampus and cerebral cortex, the predominantly expressed subunits are GluA1 and GluA2, with low levels of GluA3 and GluA4 [42] . The receptor displays high Ca 2+ and zinc permeability in the absence of the GluA2 subunit and low Ca 2+ and zinc permeability in the presence of this subunit [2] . Although receptors containing the GluA2 subunit are the most sensitive to pentobarbital, non-GluA2-containing receptors also display measurable sensitivity to this drug [43] . Therefore, we cannot rule out the possibility that, although we used a concentration of pentobarbital that should display minimal effect on GluA2-lacking AMPA receptors, there was some inhibition of the Ca 2+ /zinc-permeable GluA2-lacking receptors. The antagonist data, along with the co-immunoprecipitation data, clearly indicates that GluA2-lacking, GluA1-containing AMPA receptors are involved in the PrP C -mediated zinc uptake. One possible molecular mechanism underlying this effect is that PrP C stabilises the AMPA receptor in a zinc transport-competent location at the cell surface as evidenced by the increased surface expression of the GluA1 subunit in the presence of PrP C . Through the use of site-specific antibodies and a deletion construct, we show that the octapeptide repeats in PrP C are required for the zinc uptake. There is evidence that the four octapeptide repeats bind a single zinc ion with a Kd of 200 μM, indicating that zinc binding to PrP C is possible at the reported synaptic zinc concentrations of up to 300 μM [18] , [44] . It is thus possible that zinc binds to the octapeptide repeats with relatively low affinity, and then channels the metal to the AMPA receptor for transport across the membrane. The recent report that PrP C may be evolutionarily related to the ZIP family of zinc transporters [23] would support such a mechanism by which PrP C and AMPA receptors together facilitate zinc uptake. In the ZIP proteins, which have zinc-binding histidine-containing motifs in their extracellular N-terminal repeat sequences and a carboxy-terminal multiple-membrane-spanning domain, the zinc sensor/scavenger and membrane-transport functions are combined in the single protein; whereas in the case of PrP C and AMPA receptors, these two functions reside in different proteins. The octapeptide repeats in the glycosyl-phosphatidylinositol-anchored PrP C act as a zinc sensor/scavenger, and then transfers the metal to the transmembrane AMPA receptor for transport across the plasma membrane. Although the octapeptide repeats are required for the PrP C -mediated zinc uptake, they are not involved in the interaction with the AMPA receptor as shown by the ability of the PrPΔOct mutant to co-immunoprecipiate with the AMPA receptor subunits and the inability of zinc chelation to disrupt the PrP C -AMPA receptor interaction. However, the N-terminal polybasic region of PrP C is required for mediating the interaction with the AMPA receptor. Loss of this interaction between the two proteins appears to be critical for the PrP C -enhanced zinc uptake, as evidenced with the PrPΔN mutant and with the disease-associated mutants P101L and D177N, which all failed to co-immunoprecipitate with the AMPA receptor and to enhance zinc uptake. The N-terminal polybasic residues that are missing from the PrPΔN mutant have been implicated in several biological functions of PrP C , including endocytic trafficking and localisation to clathrin-coated pits [30] , binding of glycosaminoglycans [31] , [45] , [46] , inhibition of the β-secretase cleavage of the amyloid precursor protein [31] , binding of the amyloid-β peptide [47] and in mediating PrP C -related neurotoxicity [48] . There is discussion as to whether prion diseases are solely due to the gain of toxic function on formation of PrP Sc or whether loss of the normal function(s) of PrP C may also contribute to disease pathogenesis [14] , [15] . Our observations that zinc uptake is lost in cells expressing mutated forms of PrP C associated with the human prion diseases CJD, GSS and familial fatal insomnia, and in persistently scrapie-infected cells, lend support to the latter hypothesis. Consistent with this observed reduction in zinc uptake in the scrapie-infected cells, the zinc content of brains from scrapie-infected mice was reduced by >70% [34] , and in the frontal cortex of sporadic CJD cases the zinc content was decreased compared with controls [33] , providing additional evidence that upon conversion to PrP Sc neuronal uptake of zinc may be compromised. It has been suggested that some features of the neurological illness associated with inherited PrP C mutations may be attributable to a loss of PrP C neuroprotective function [49] . In this context, it is interesting to note that the PG14 mutant associated with familial CJD [35] , which had impaired neuroprotective activity in transgenic mice [50] , was ineffective in enhancing zinc uptake. The role we have described here for PrP C in mediating neuronal zinc uptake may also impact on another neurodegenerative disorder. Alzheimer's disease (AD) is characterised by the extracellular accumulation of the neurotoxic amyloid-β peptide [51] . Zinc promotes the aggregation of amyloid-β into toxic oligomeric forms [52] . In an AD mouse model, synaptic zinc was shown to increase insoluble amyloid-β and its deposition in plaques [53] . Synaptic zinc favours the attachment of amyloid-β oligomers to the N-methyl- D -aspartate receptor, mediating their excitotoxicity [54] , and PrP C itself is a high-affinity receptor for amyloid-β oligomers [55] . Thus, the reduction in PrP C in the brain in AD [56] would result in decreased zinc uptake, thereby increasing zinc in the synaptic cleft, which in turn would promote amyloid-β aggregation and synaptic targeting, potentially contributing to the neurodegeneration in AD. In conclusion, using zinc-specific fluorescent dyes and selective receptor antagonists, we have shown for the first time that PrP C enhances the uptake of zinc into neuronal cells through AMPA receptors, with a subsequent downstream effect on the activity of intracellular protein tyrosine phosphatases. The octapeptide repeats in PrP C are critical for this zinc uptake, and PrP C interacts with both GluA1 and GluA2 subunits of AMPA receptors through its N-terminal polybasic region. In addition, in cells expressing mutants of PrP C associated with human prion diseases or in scrapie-infected cells, this PrP C -mediated zinc uptake is lost, raising the possibility that loss of this function may in part contribute to the pathogenesis of prion disorders and other neurodegenerative diseases. Thus, we have provided the molecular framework underpinning the mechanism by which PrP C is involved in neuronal zinc uptake, and have introduced a new facet to prion biology. Cell culture and construction of prion protein mutants Cell culture, preparation of rat primary hippocampal neurons and construction of PrP C mutants is described in Supplementary Methods . Zinc was routinely administered to the cells as ZnCl 2 in the presence of 10% FCS to provide appropriate physiological ligands (albumin and histidine) for the zinc to complex to. When the cells had reached confluency, they were collected into PBS (1.5 mM KH 2 PO 4 , 2.7 mM Na 2 HPO 4 , 150 mM NaCl, pH 7.4), pelleted and resuspended in lysis buffer (10 mM Tris/HCl, pH 7.8, 0.5% (w/v) sodium deoxycholate, 0.5% (v/v) Nonidet P-40, 100 mM NaCl, 10 mM EDTA, supplemented with complete protease inhibitor cocktail (Sigma, P8340)). The protein content of each lysate was determined using bicinchoninic acid with BSA as standard. Measurement of zinc uptake using Zinpyr-1 or Newport Green Cells were cultured overnight in 10% FCS-containing DMEM. For staining with Zinpyr-1, following adherence, the cells were exposed to 10% FCS-containing media supplemented with ZnCl 2 . The media was removed, the cells were washed three times with PBS (containing Ca 2+ and Mg 2+ ) before 10 μM Zinpyr-1 (a gift from Dr A. Favier, Université Joseph Fourier, Grenoble, France) in 50 mM PIPES, 100 mM KCl, pH 7, was delivered to the cells for 30 min at 37 °C. The cells were washed a further three times with PBS (containing Ca 2+ and Mg 2+ ), then 50 mM PIPES, 100 mM KCl, pH 7, was added and the Zinpyr-1 fluorescence measured on a Synergy HT (Bio-Tek; 480 nm excitation and 530 nm emission wavelengths). At the end of the time period, the cells were fixed in 70% ethanol at room temperature for 5 min and the adherent monolayers stained with the DNA-binding fluorochrome Hoescht 33342 (8.8 μM). Once dry, the fluorescence was measured (350 nm excitation and 450 nm emission wavelengths) to determine the cell number and enable standardisation of the Zinpyr-1 fluorescence. For staining with Newport Green, the cells were loaded with 5 μM Newport Green (Invitrogen, Paisley, UK) delivered in 10% FCS media. After 30 min, the dye was replaced with 10% FCS-containing media supplemented with ZnCl 2 . The fluorescence was immediately measured (480 nm excitation and 530 nm emission wavelengths) for up to 30 min. Finally, the cells were fixed in 70% ethanol and stained with Hoescht 33342 as described above. Where indicated, the AMPA receptor antagonists CNQX (Ascent Scientific, Bristol, UK), IEM-1460 (Sigma) or sodium pentobarbital (Euthatal, Marial Animal Health Ltd, Harlow, Essex, UK) were included in the incubations. To determine whether PrP C promoted intracellular zinc retention, cells were pre-loaded with 32 μM ZnCl 2 in 10% FCS-containing medium for 1 h. Newport Green (5 μM) was added for a further 30 min to label the zinc taken up into the cells. At the end of this incubation, the medium was removed, fresh 10% FCS medium added and the level of fluorescence within the cells immediately quantified. For each time point over the course of the experiment, the old medium was removed and fresh medium applied before measurement to ensure that any fluorescence measured was derived from the cells and not the associated medium. As before, the cells were fixed in 70% ethanol and stained with Hoescht 33342 as described above. SDS–PAGE and western blot analysis Samples (containing 15 μg of total protein) or immunoprecipitates were resolved by electrophoresis through either 14.5 or 10% polyacrylamide gels [31] . For western blot analysis, resolved proteins were transferred to Hybond-P poly(vinylidene) difluoride membrane (Amersham, Little Chalfont, UK). The membrane was blocked by incubation for 1 h with PBS containing 0.1% (v/v) Tween 20 and 5% (w/v) dried milk powder. Incubations with primary antibodies, including 3F4 and 6D11 (both from Eurogentec Ltd, Southampton, UK), SAF32 (Bertin Pharma, France), 6H4 (Celtic Diagnostics, Dublin, Eire), 8H4 (Alicon AG, Switzerland) against PrP C , an antibody against GluA1 (Abcam, Cambridge, UK) and an antibody against GluA2 (UCDavis/NIH NeuroMab Facility), Shadoo (Santa Cruz, CA, USA), DDC39 (anti-Dpl antibody was a generous gift from S. Lehmann (Montpellier, France)) and peroxidase-conjugated secondary antibodies were performed for 1 h in either the same solution (for antibody 3F4) or 2% BSA in PBS containing 0.1% (w/v) Tween 20 (for all other antibodies). Bound peroxidase conjugates were visualised using an enhanced chemiluminescence detection system (Amersham) and recorded using Fujifilm LAS-3000. All western blots were repeated a minimum of three times. RNA interference studies An siRNA specific for murine and rat PrP C or human LRP1 (ON-TARGETplus SMART-pool, Dharmacon (Thermo Fisher Scientific Biosciences, Northumberland, UK)) or negative control siRNAs (ON-TARGETplus Non-Targeting Pool, Dharmacon) were as detailed in ref. [28] 28. Cells were washed twice with PBS (containing Ca 2+ and Mg 2+ ) and a 2 μM SMART-pool siRNA solution (Dharmacon) delivered as a complex with DharmaFECT-1 (Dharmacon; for SH-SY5Y and N2a cells) or DharmaFECT-3 (Dharmacon; for rat primary hippocampal neurons) transfection reagent in serum-free media. After 5 h, the serum-free media were replaced with 10% FCS-containing DMEM and the cells left for 48 h, and then either lysed for western blot analysis or stained with Newport Green. Co-immunoprecipitation Brain tissue from 75-day-old wild-type or PrP −/− 129/P2 mice was homogenised under ice-cold conditions for 10 s in 50 mM Tris/HCl, 2 mM EDTA, 150 mM NaCl, 1% (w/v) CHAPSO, pH 7.5. The P101L mice were 29 days old [57] , D177N(M128) mice were 30–54 days old and the D177N(V128) mice were 36 days old [58] . All samples were pre-cleared using (0.25% w/v) protein A or protein G Sepharose for 30 min at room temperature. The Sepharose was pelleted and the supernatant incubated with the relevant antibody (6H4 for PrP, GluA1, GluA2 and control rabbit anti-mouse IgG, or no antibody for the bead-only control) overnight at 4 °C. The antibody–antigen complexes were pelleted using either protein A or protein G Sepharose (0.5% w/v) for 1 h at room temperature and washed with 10 mM KOAc, 1.5 mM MgCl 2 , 75 mM sodium citrate, pH 6.4. The immunoprecipitates were then analysed by western blotting. For the chelation studies, 20 μM TPEN was included in all buffers, and washes used in the protocol once homogenisation had occurred. Fluorescence microscopy Cells were seeded onto coverslips and grown to 50% confluence. The cells were pre-loaded with Newport Green for 30 min before exposure to Zn 2+ for an additional 30 min. Cells were then fixed with 4% (v/v) paraformaldehyde in PBS for 15 min. PrP C was detected using antibody 3F4 with AlexaFlour 594 donkey anti-mouse secondary antibody (Invitrogen, Scotland). Nuclear counterstaining was performed using Hoescht 33342 for 5 min before mounting on slides using Fluoromount-G (SouthernBiotech) mounting medium. For primary neurons, cells were fixed in 4% (v/v) paraformaldehyde in PBS for 10 min, and then permeabilised with 0.1% Triton X-100 for 20 min. PrP C was detected using antibody 6H4 (Prionics AG, Switzerland) with AlexaFlour 488 donkey anti-mouse secondary antibody (Invitrogen). Individual cells were visualised using a DeltaVision Optical Restoration Microscopy System (Applied Precision Inc., USA). Data were collected from 30- to 40 0.1-μm thick optical sections, and three-dimensional data sets were deconvolved using the softWoRx programme (Applied Precision Inc.). The presented images represent individual Z -slices corresponding to the middle of the cell. Surface biotinylation and zinc-stimulated endocytosis of PrP C Cells were incubated for 1 h at 4 °C with 0.5 mg ml −1 Biotin sulfo-NHS (Sigma-Aldrich). Immunoprecipitation of biotin-labelled GluA1 was carried out to determine the surface expression of GluA1. Alternatively, following surface biotinylation, cell monolayers were incubated at 37 °C in the presence of Zn, with 20 μg ml −1 RAP or LRP1 siRNA as inhibitors of endocytosis [28] , and then treated with trypsin to remove any biotinylated PrP C remaining at the cell surface, with any internalised PrP C being protected from digestion. Measurement of tyrosine phosphatase activity Confluent cell monolayers were collected into PBS. Samples were then pelleted and resuspended in lysis buffer (20 mM Tris/HCl, 150 mM NaCl, 1% (v/v) Nonidet-P40, pH 7.4) supplemented with complete protease inhibitor cocktail (Sigma, P8340). Whole-brain homogenate (120 mg ml −1 wet weight in PBS, 0.5% NP-40 (v/v), 0.5% sodium deoxycholate (v/v) and protease cocktail inhibitor (Roche Diagnostics GMbH, Germany)) was prepared from 40-week-old wild-type 129/P2 and 129/P2 PrP −/− mice under ice-cold conditions, followed by centrifugation at 100,000 g for 1 h at 4 °C. The resulting supernatant was collected and analysed for enzyme activity. The cell lysates and whole-brain homogenate were analysed using the Tyrosine Phosphatase Assay System (Promega, V2471) according to the manufacturer's instructions. Statistical analysis All cell analyses were subject to Kruskal–Wallis non-parametric one-way analysis of variance, with analyses of the Newport Green kinetic data being carried out on the terminal fluorescence value for each measurement within the triplicate data set. The brain sample data were analysed by parametric independent Student's t -test. How to cite this article: Watt, N.T. et al . Prion protein facilitates uptake of zinc into neuronal cells. Nat. Commun. 3:1134 doi: 10.1038/ncomms2135 (2012).